High mobility explains demand sharing and enforced cooperation in egalitarian hunter-gatherers ‘Simple’ hunter-gatherer populations adopt the social norm of ‘demand sharing’, an example of human hyper-cooperation whereby food brought into camps is claimed and divided by group members. Explaining how demand sharing evolved without punishment to free riders, who rarely hunt but receive resources from active hunters, has been a long-standing problem. Here we show through a simulation model that demand-sharing families that continuously move between camps in response to their energy income are able to survive in unpredictable environments typical of hunter-gatherers, while non-sharing families and sedentary families perish. Our model also predicts that non-producers (free riders, pre-adults and post-productive adults) can be sustained in relatively high numbers. As most of hominin pre-history evolved in hunter-gatherer settings, demand sharing may be an ancestral manifestation of hyper-cooperation and inequality aversion, allowing exploration of high-quality, hard-to-acquire resources, the evolution of fluid co-residence patterns and egalitarian resource distribution in the absence of punishment or warfare. ‘Simple’ hunter-gatherers [1] are found in Africa, Southeast Asia and South America, predominantly egalitarian [2] , monogamous, highly mobile, and lack resource storage and wealth accumulation [1] , sharing food with related and unrelated group members to an extent not observed in other human populations or other species [3] . This is often explained by ‘demand sharing’ [4] , the social norm by which individuals in possession of highly coveted resources (such as meat) are forced to share food with all other group members (including free-riding individuals who rarely hunt). Meat butchering and distribution are done as a rule by individuals other than the hunter, whose family does not necessarily get a bigger share than other families [5] . Together, such rules of sharing can be seen as a prior social agreement establishing a cost to non-compliance [6] , with anecdotal evidence from some hunter-gathering groups suggesting the mocking and ridiculing of stingy individuals [2] . Food sharing is crucial to hunter-gatherers who heavily rely on high-quality but unpredictable and hard-to-acquire resources [3] . The dependence on food transfers as a buffer to the uncertainty of food acquisition and limitations to long-term storage imply a highly egalitarian social organization and an absence of individual ownership of resources (including game) in simple hunter-gatherer societies, in contrast to more stratified agriculturalists, pastoralists and ‘complex’ hunter-gatherers [1] , [2] , [4] . Demand sharing, by opposing the presence of non-sharers (loners) and enforcing food sharing and collective resource ownership, has been widely recognized as a fundamental adaptation in simple hunter-gatherers [2] , [3] , [4] , [5] , [7] , [8] , [9] , [10] , [11] , [12] . However, explaining how demand sharing can resist the spread of non-hunters (free riders), who demand and receive food despite not hunting (or hunting at low frequencies), remains a long-standing problem. Moreover, such non-hunters have been observed in many populations [7] , [8] without prompting explicit forms of punishment (such as exclusion from camps or from food sharing). The free-rider problem faced by extant hunter-gatherers resembles the ones addressed by economic games such as the Public Goods Game [13] , N-Player Prisoner’s Dilemma, or Hawk-Dove Game [14] among others, where pay-offs to general cooperation (‘everybody hunts’) are higher than pay-offs to general defection (‘nobody hunts’), but lower than pay-offs to free riders living among co-operators (‘everybody hunts but me’) [7] , [8] . However, current economic games do not reproduce the specific social, ecological and life history characteristics that define the hunter-gatherer lifestyle, such as enforced food sharing, an intricate life cycle characterized by long growth and senescence stages (which imply large numbers of low-producing individuals in addition to free riders, such as pre-adults and older hunters) [15] , and a niche characterized by high-quality but unpredictable and hard-to-acquire resources [16] , which together tell apart human hunter-gatherers from earlier hominins and closely related African apes [17] , [18] . Here we present an agent-based model that realistically simulates hunter-gatherer populations living in an unpredictable environment, and then compare the results with data from real hunter-gatherers. Our results indicate that mobility is a key factor in maintaining the cooperative system of demand sharing in hunter-gatherers. We show that families that keep moving between camps and practice demand sharing with other unrelated families can prevent the spread of free riders in populations, and therefore survive despite the unpredictability of hunting returns. In contrast, both loner families (that do not share food) and sedentary demand sharers fail to survive in similarly unpredictable environments. We argue that demand sharing may be an important ancestral manifestation of hyper-cooperation in humans, allowing hunter-gatherers, through a combination of egalitarian resource distribution and high mobility, to explore high-quality but hard-to-acquire resources, to evolve fluid co-residence patterns and to maintain high levels of cooperation in the absence of punishment or warfare. Agent-based simulation of demand sharing To investigate the conditions that led to the evolution of demand sharing in humans, we present an agent-based model with 15 parameters incorporating key features of the hunter-gatherer lifestyle (see Methods for full details). Each simulated agent represents the combined features of all individuals constituting a monogamous, nuclear family unit (adult male, female and dependent offspring) rather than a single individual, so that its energy production represents meat production by a male hunter (parameter k , or value of a kill); energy consumption reflects the metabolic costs of the male, female and all offspring (DCs, daily maintenance costs); hunting implies an additional cost (HCs, hunting costs). The survival curve of agents is modelled after empirical survival curves derived from hunter-gatherer groups ( a and b , age-specific mortality coefficients); agent fertility is modelled after female fertility, reflecting reproductive constraints imposed on families by monogamy (no reproduction before the age of 15 years and a maximum of one offspring per year). Agents (the whole family unit) die when their energy balance reaches zero and reproduce only if the offspring survives to age 15 years (age, age at independence), which depends on the parental agent maintaining sufficient energy levels during offspring development (RepT, reproductive threshold). Storage is only possible in the form of body fatness and has an upper limit corresponding to 30 days of survival ( f , maximum energy storage). Family units can move at a cost (MCs, movement costs) around 20 possible locations (location number), reflecting the high mobility of hunter-gatherers as a response to the energy income obtained at a given location (thresh, movement threshold). Propensity to hunt is heritable ( w , daily probability or propensity to hunt) but subject to random mutation ( m , mutation rate), with each agent being either an active hunter (with propensity to hunt in the interval w =(0.75–1.00)), or a free rider ( w ≤0.1). On a day a hunter goes on a hunting trip (with probability w ), its daily probability of hunting success will be the product of: age-dependent hunting ability based on empirical curves of calorie production in male hunters [10] (peak, age at peak hunting ability), number of hunters in the same location to account for density effects on hunting productivity (dens, density-dependent effects) and a varying probability of the presence of game in a given camp ( p , environmental quality). We simulated the population dynamics of agents daily and over 1,500 years, following the algorithm presented in Fig. 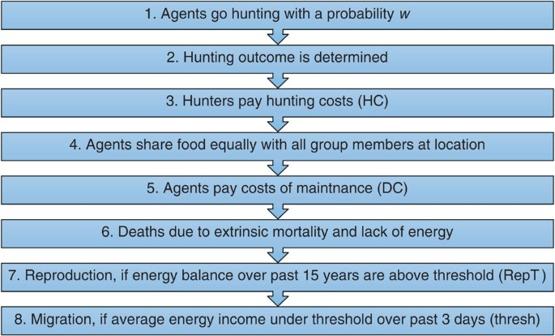Figure 1: Diagram showing the main steps of the model simulation. Diagram shown is for mobile demand-sharing populations. When agents are loners step 4 is omitted, and when agents are sedentary step 8 is omitted. 1 , and collected demographic data at the end of simulations (see Methods for definition of parameters, Supplementary Methods and Supplementary Figs 1 to 16 for parameter range exploration, and Supplementary Table 1 for intervals tested and used values). Figure 1: Diagram showing the main steps of the model simulation. Diagram shown is for mobile demand-sharing populations. When agents are loners step 4 is omitted, and when agents are sedentary step 8 is omitted. Full size image Survival in harsh environments requires demand sharing We first compared the long-term dynamics of simulated populations under two conditions: agents required to share any produced food with all camp members (demand sharing) and agents consuming all they produced without sharing (loners). We compared survival (time to collapse) of demand sharers and loners, both in separate or the same simulations. We obtained similar results in both scenarios (as expected, as loners neither give nor receive food from other agents); however, as by definition demand sharing prevents the presence of loners [2] , [4] , we present the results from separate simulations. Results show that populations of demand sharers were highly resilient and likely to avoid extinction over 1,500 simulated years, except under the harshest environmental conditions (when environmental quality p , or the daily probability of the presence of game at a given location, was set at a fixed value of P =0.5 or lower, or varying between P= (0.2–1.00) or lower; Fig. 2 and Supplementary Figs 1 and 2 ). In contrast, loners were able to survive only under more favourable environmental conditions (fixed P ≥0.8, or variable P ≥(0.4–1.00)). Crucially, under values of environmental quality between the two extremes above (that is, fixed P= 0.6 and P= 0.7, or variable P= (0.3–1.00)), demand-sharing populations typically survived to the end of simulations, while loner populations quickly went extinct. Such intermediate values of environmental quality p correspond to harsh conditions, resulting in a rate of daily hunting success (the product of environmental quality on that day, agent-specific hunting ability and dens) of only 33% for each agent, closely matching the average rate in real hunter-gatherers (28% for Hadza, 27% for!Kung and 10–30% for Efe; Table 1 ). Enforced food sharing therefore saves adults and their offspring from food shortage in 2 out of every 3 days. The results above demonstrate the importance of the demand-sharing strategy to populations of hunter-gatherers usually facing environments characterized by high unpredictability. 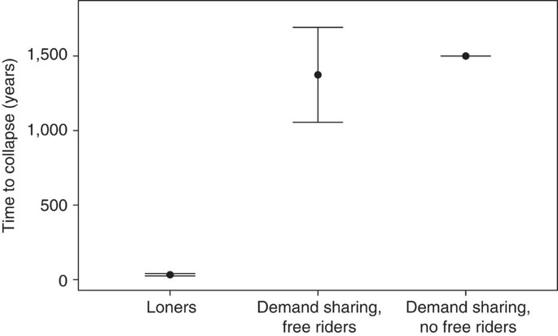Figure 2: Time to collapse of simulated populations. Populations shown are loners, demand sharing with free riders and demand sharers without free riders. Environmental quality (p) was variable withpin (0.3–1). Mobile populations of demand-sharing populations (with or without free riders) survive for the 1,500 years of the simulation, whereas mobile loners quickly collapse. Results shown are means and s.d. for ten replicates. Figure 2: Time to collapse of simulated populations. Populations shown are loners, demand sharing with free riders and demand sharers without free riders. Environmental quality ( p ) was variable with p in (0.3–1). Mobile populations of demand-sharing populations (with or without free riders) survive for the 1,500 years of the simulation, whereas mobile loners quickly collapse. Results shown are means and s.d. for ten replicates. Full size image Table 1 Movement, camp size and success rate per hunt in simulated (demand sharing) and real hunter-gatherer populations. Full size table Mobile hunter-gatherers avoid the spread of free riders Next we investigated the conditions under which the demand-sharing strategy would be able to resist the challenge posed by the presence of free riders (agents who still demand resources but have low propensity to hunt). Our simulations investigated demographic trends within demand-sharing populations, with free riders being allowed to appear by mutation. Simulations show that when demand-sharing agents are sedentary (meaning that they are not allowed to move to new locations), free riders increase in number within populations, active hunters decrease in number and populations go extinct due to overall low productivity ( Fig. 3 ). However, an important result is that when both active hunters and free riders are allowed to move from camps where net energy income is low (either due to low environmental quality or to the presence of a number of non-productive free riders), populations do not collapse, active hunters remain a significant fraction of the demand-sharing populations and free riders make up a small but persistent fraction of groups (time average of 10%; Supplementary Fig. 17 ) in the absence of any form of direct punishment to free riders ( Fig. 3 ). Active hunters experience larger camp sizes and move more frequently between camps than free riders ( Supplementary Figs 18 and 19 ), as only they incur HCs and hence more often reach the low-energy-intake threshold that triggers movement to other camps. In summary, free riders accelerate the collapse of sedentary demand-sharing populations, but do not prevent the survival of mobile demand-sharing populations, irrespective of environmental quality (see Fig. 3 and Supplementary Figs 1 and 2 ). 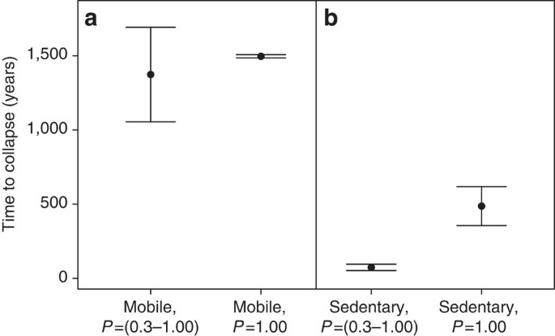Figure 3: Time to collapse of simulated populations of mobile versus sedentary demand sharers. (a) Mobile demand sharers with free riders and (b) sedentary demand sharers with free riders as a function of environmental quality (p). Environmental quality (p) was simulated in two different scenarios: withpin (0.3–1) andp=1. Mobile demand-sharing populations with free riders survive for the 1,500 years of the simulation, whereas sedentary populations with free riders quickly collapse even when environment is ‘ideal’ (p=1). Results shown are means and s.d. for ten replicates. Figure 3: Time to collapse of simulated populations of mobile versus sedentary demand sharers. ( a ) Mobile demand sharers with free riders and ( b ) sedentary demand sharers with free riders as a function of environmental quality ( p ). Environmental quality ( p ) was simulated in two different scenarios: with p in (0.3–1) and p= 1. Mobile demand-sharing populations with free riders survive for the 1,500 years of the simulation, whereas sedentary populations with free riders quickly collapse even when environment is ‘ideal’ ( p= 1). Results shown are means and s.d. for ten replicates. Full size image Simulated mobility rates match real hunter-gatherer data As a test for the model, we investigated the match between frequency of between-camp movement, population per camp and daily probability of hunting success in simulated demand-sharing populations and real hunter-gatherer populations ( Table 1 and Fig. 4 ). Predicted movement frequency (5.2 days between moves) is at the higher end of the real hunter-gatherers range, but close to the observed frequency in groups such as the Ache, Punan and Hiwi (6.3, 8.1 and 9.1 days between moves, respectively). As we proposed that high mobility is a condition for the maintenance of demand-sharing populations, we investigated the values of days between moves compatible with the survival of simulated populations. The results revealed a striking match to the observed frequencies of movement in real hunter-gatherer groups ( Fig. 4 ). Our model predicts the survival of demand-sharing groups with free riders when movement rates vary between 5 and 30 days between moves, interval that includes 11 of the 12 demand-sharing groups in Table 1 . Together, the results show that the combination of compulsory food sharing and movement triggered by insufficient energy income is a superior strategy both to the mobile, non-sharing strategy of loners and to a sedentary, sharing strategy, as it deals more efficiently with the effects of unpredictability of food resources and significantly reduces the probability of population collapse by using mobility as a free-rider avoidance mechanism. 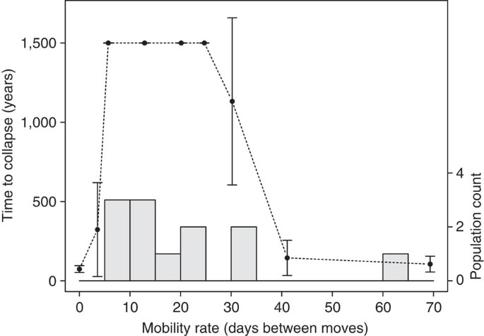Figure 4: Distribution of mobility rates in simulated and real hunter-gatherer populations. The graph shows time to collapse of simulated demand-sharing populations with free riders as a function of mobility rate (black circles with s.d. bars; left axis) and number of real hunter-gatherer groups according to mobility rate (grey bars; right axis). We obtained a series of populations differing in mobility rate (days between moves) by varying the parameter thresh. Populations with mobility rates between ~5–30 days per move mostly survive to the end of simulations. Survival decreases with higher or lower mobility rates. Histograms are based on the 12 demand-sharing hunter-gatherer groups listed inTable 1. Bars represent five-unit intervals of days per move. Five to 10 days per move: Punan, Ache and Hiwi. Ten to 15 days per move: Semang, Agta and Hadza. Fifteen to 20 days per move: Aeta. Twenty to 25 days per move: Gwi and Baka. Thirty to 35 days per move: Efe and Mbuti. The!Kung show extremely low mobility rates (63.4 days between moves). As reported by Kelly21, the mobility of the!Kung from the Kalahari Desert is restricted by access to wells. Figure 4: Distribution of mobility rates in simulated and real hunter-gatherer populations. The graph shows time to collapse of simulated demand-sharing populations with free riders as a function of mobility rate (black circles with s.d. bars; left axis) and number of real hunter-gatherer groups according to mobility rate (grey bars; right axis). We obtained a series of populations differing in mobility rate (days between moves) by varying the parameter thresh. Populations with mobility rates between ~5–30 days per move mostly survive to the end of simulations. Survival decreases with higher or lower mobility rates. Histograms are based on the 12 demand-sharing hunter-gatherer groups listed in Table 1 . Bars represent five-unit intervals of days per move. Five to 10 days per move: Punan, Ache and Hiwi. Ten to 15 days per move: Semang, Agta and Hadza. Fifteen to 20 days per move: Aeta. Twenty to 25 days per move: Gwi and Baka. Thirty to 35 days per move: Efe and Mbuti. The!Kung show extremely low mobility rates (63.4 days between moves). As reported by Kelly [21] , the mobility of the!Kung from the Kalahari Desert is restricted by access to wells. Full size image Food transfers extend lifespans in simulated demand sharers Our simulation model reproduces the known fact that active hunters produce a significant lifetime surplus of energy ( Fig. 5 ) shared with low and non-producers. Low producers include non-hunters (free riders), immature individuals undergoing extended growth and development [16] , and older or ‘post-productive’ individuals (whose calorie production at older ages drops below consumption levels). Owing to energy transfers from peak-hunting individuals, simulated life expectancy at the age of independence (15 years) is higher in demand-sharing groups than among loners ( Supplementary Table 2 ). 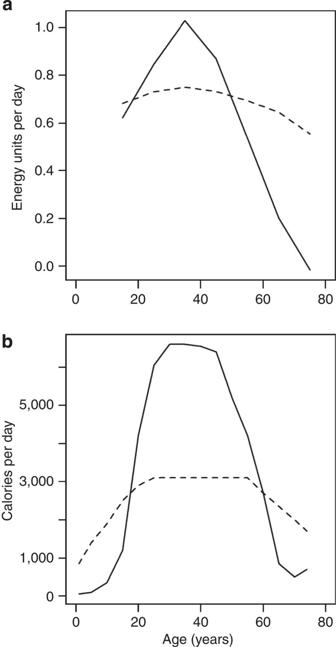Figure 5: Energy production and consumption in simulated and real hunter-gatherers. (a) Age-specific daily energy production (solid lines) and consumption (dashed lines) from age 15 years in simulated demand-sharing agents. (b) Real data for human hunter-gatherers (real production and consumption curves adapted from ref.16, is a mean from Ache, Hadza and Hiwi male production). Figure 5 also highlights the decline in hunter productivity below maintenance levels at around age 50 years. At that point, adults also become dependent on food transfers. Accordingly, life expectancy at age 50 years in the simulated demand-sharing population (9.1 years) was close to that observed in the Agta (10.8 years), whereas in simulated loners (3.3 years) values were more similar to observed life expectancy in chimpanzees (4.5 years). As chimpanzees do not depend on food sharing after weaning and are in this sense loners (despite not hunting at high frequencies), our results suggest that the evolution of demand sharing and generalized food provisioning may have occurred early in the Homo lineage and may have led to fundamental changes in human life history from an ape-like to a hominin-like pattern, including an extended period of pre-adult dependence and longer lifespans. Figure 5: Energy production and consumption in simulated and real hunter-gatherers. ( a ) Age-specific daily energy production (solid lines) and consumption (dashed lines) from age 15 years in simulated demand-sharing agents. ( b ) Real data for human hunter-gatherers (real production and consumption curves adapted from ref. 16 , is a mean from Ache, Hadza and Hiwi male production). Full size image By setting our model in the specific socio-ecological context of hunter-gatherers, with the realistic requirements that resources needed for survival are obtained from the environment, we have shown that demand-sharing populations can resist collapse due to the spread of free riders solely through free movement of family units around camps, a solution that simultaneously solves the problem of resource uncertainty [10] , [11] . Our simulations demonstrate the compatibility of demand sharing with the continuous spatial mobility of both active hunters and free riders. Other proposals such as the ‘Walk Away’ [19] model have concluded that spatial mobility accelerates the evolution of cooperation through positive assortment of cooperators and resulting avoidance of free riders, but this solution is associated with a drastic reduction in mobility rates. Positive phenotypic assortment has also been evoked to explain between-camp differences in levels of cooperation in a Public Goods Game among Hadza hunter-gatherers [20] , with highly cooperative Hadza individuals living together in certain camps and thereby ‘excluding’ free riders. The main problem with such proposals is that phenotypic assortment is not compatible with the observed high mobility and freedom of movement of hunter-gatherers [1] , [21] , [22] , [23] , [24] . For this reason, they do not show how positive phenotypic assortment could exclude free riders (who are in principle as mobile as active hunters) from ‘cooperative’ camps, without explicit punishment. The finding of the Walk Away model that high cooperation, here exemplified by demand sharing, would be associated with reduced between-camp mobility, is also contradicted by evidence from hunter-gatherer groups, who are highly mobile [1] ( Table 1 ). In contrast, our model requires neither permanent assortment nor a reduction of mobility once demand sharing is established. On the contrary, it requires constant movement between camps and predicts a collapse of demand-sharing populations when agents are sedentary ( Fig. 3 ). In fact, ethnographic studies have shown that demand sharing does break apart when hunter-gatherer populations are forced to settle [3] . Finally, the combination of high-cooperation and mobility was derived in our simulations without the postulation of any form of punishment or limitations on the mobility of free riders, in agreement with the evidence from real hunter-gatherer groups. The main evolutionary implication of our model is that demand sharing may have originated early in the hominin lineage when large-game hunting became the major source of calories. This transition would have depended on high mobility, both to allow access to high-value but unpredictable and spatially sparse meat sources [17] , [18] , and to allow active hunters to avoid camps temporarily hosting free riders. This scenario explains the maintenance and viability of enforced food sharing among unrelated individuals without the need for explicit mechanisms of reciprocity and first- and second-order punishment of non-hunting free riders [25] , [26] . Although the evolution of more sophisticated punishment mechanisms may have been facilitated once the simpler avoidance-by-movement mechanism was established, our model suggests that they were not necessary for the origin of demand-sharing groups. An important implication for human life history is that the predicted reduction of later life mortality as a result of demand sharing may also have led to larger cohorts of individuals surviving to older ages, and thus provided the selective context for the evolution of grandmothering [27] . Furthermore, the movement of nuclear families as a whole between camps is compatible with the evolution of bisexual philopatry (or dispersal of both sexes) characteristic of humans, in contrast to the patrilocal and matrilocal residence patterns of apes [28] . Finally, our proposed scenario for the evolution and maintenance of the hunter-gatherer lifestyle does not require intergroup competition and cultural group selection [29] as conditions for intragroup cooperation. Our proposal is therefore compatible with low levels of warfare among African hunter-gatherers [30] and derives cooperative behaviour, egalitarianism and non-kin extended social networks [20] from selective pressures at the individual level [31] . Model design We investigated the origin and consequences of demand sharing through an agent-based model incorporating key features of the hunter-gatherer lifestyle: hunting, moving, sharing, reproducing and ageing. We use a walk-away (or win-stay/lose-shift) rule to determine agent movement [19] , [32] , [33] . Each simulated agent represents the combined features of all individuals constituting a monogamous, nuclear family unit (adult male, female and dependent offspring), so that its energy production represents meat production by a male hunter. Energy consumption reflects metabolic costs of male, female and dependent offspring. Hunting and moving to other locations also involve costs. At age 15 years, surviving offspring become independent agents [34] , [35] . We simulated the existence of different agent strategies: loners (agents that actively hunt but do not share resources outside the nuclear family) and demand sharers (agents that are forced to share any food obtained by hunting with other agents present in the same camp or location). Demand-sharing populations were simulated in three different ways: only mobile active hunters, mobile active hunters and free riders (who have low propensity to hunt but nonetheless share resources brought to the camp by active hunters), and sedentary populations of active hunters and free riders. Food is modelled as a high-quality and unpredictable resource, such as meat from game, returned after hunting. Each agent has a level of energy increased by feeding and reduced by MCs, HCs and DCs. Agents can store a maximum number of units of energy as body fat corresponding to 30 days of maintenance costs or ability to survive without food if they are not hunting or moving. Agents die if their energy falls below 0 units. We also added background daily mortality probability (as in real human populations, increasing after independence). Agent longevity represents either adult male or female survival as we assume no significant dimorphism in adult survival. Agent reproduction reflects fertility patterns in a monogamous population (no reproduction before the age of 15 years, maximum of one offspring per year). Reproduction is recorded only if offspring survives to age 15 years (which depends on energy levels maintained during offspring development). Offspring inherit the same hunting phenotype as their family unit. In some simulations, free riders (non-hunters) are introduced through a mutation in hunting propensity. Agents can move throughout a landscape with 20 possible locations (representing camps). Agents move to randomly selected locations independently of anyone else leaving. Agents move in response to their net energy income over the last 3 days at their current location, moving if its mean value drops below a threshold. In simulations where agents do not share with other agents (loners), each agent’s energy balance is increased by the daily amount of energy that they produced. In simulations where agents share, successful hunters at a location equally distribute pooled resources among all agents in that location (irrespective of whether an agent hunted or was successful in a hunt). Only individuals who hunted incur the energy cost of hunting (irrespective of success). Hunting ability of real hunter-gatherers changes with age due to the high level of skill, knowledge and strength required to hunt [5] . Studies have reported an initial learning period during which production is low, and age-related senescence causes a reduction in productivity [16] , [36] . To reflect this, we model the probability that an agent successfully hunts as a function of age-dependent ability, peaking at age 35 years [16] , the location-based probability of finding game and the number of other hunters in that location. Simulations Simulations start with 100 agents, with an age structure roughly similar to that of a traditional society [37] . Initial energy is distributed between 50% and 70% of the maximum energy storage limit. All agents who are old enough are assumed to be at least 365 days past their last reproduction (so that this does not restrict initial reproduction). Any agent in the initial population is removed from the analysis. Agents are distributed among half of the possible locations but are free to move, except in sedentary populations where they are randomly distributed among all possible locations. Simulations are run to model life on a daily basis for 1,500 years. For each parameter combination, ten independent replicates are run. Owing to density-dependence effects, populations rarely reached 250 individuals. Simulations were run using Matlab R2012a [38] . Figures were produced in R [39] using the packages lattice [40] , ggplot2 (ref. 41 ), gridExtra [42] , plyr [43] and reshape [44] . Model parameters Definitions and range of tested values of each of the 15 model parameters and parameter explorations are presented in Supplementary Table 1 , Supplementary Methods and Supplementary Figs 1 to 16 . Criteria for selection of parameter values (parametrization) were based on our aim of simulating a hunter-gatherer lifestyle and are discussed below. Environmental quality ( p ) is a measure of daily probability of presence of game at a given location. p was set as either fixed or variable depending on the scenario. Variable scenarios allow us to test the effect of unpredictability of environments. In the variable scenarios, p in each location changed every 5 days, with a new value being chosen independently at each location and randomly from a uniform distribution. We ran simulations exploring a range of fixed and variable values of environmental quality ( Supplementary Methods and Supplementary Figs 1 and 2 ) and evaluated their effect on the survival of the four types of populations (loners, mobile demand sharers with free riders, mobile demand sharers without free riders and sedentary demand sharers). Active hunters in demand-sharing populations have a daily propensity to hunt w fixed throughout their lifetime and drawn from a uniform distribution between w =0.75 and w =1 at the age of independence. Free riding are introduced through a mutation in hunting propensity, with their w chosen from a uniform distribution between w =0 and w =0.1 at the time of independence. Free riders are therefore demand sharers (that is, they participate in the sharing pools) with low propensity to hunt. We used the discrete intervals of w described above to force the introduction of a free rider every time a mutation occurred. Agents who are active hunters produce offspring who are active hunters, except if a mutation takes place; free riders produce offspring who are free riders. Mutation rate in hunting propensity was set at m =0 (scenarios without free riders) or m =0.005 (scenarios with free riders). Explorations of parameter m are shown in Supplementary Methods and Supplementary Figs 3 and 4 . The curve of age-specific hunting ability was defined as huntab=0.9 × exp(−(age−peak) × 365)) 2 /(2 × 7,300 2 )), with age in days, and produces a peak value of 0.9 in hunting ability at age 35 years to match empirical evidence [16] , [36] . The hunting ability function was based on production curves for real hunter-gatherers [16] . However, we have varied the age of peak production to explore the effect of this parameter in the model ( Supplementary Methods and Supplementary Figs 5 and 6 ). Density-dependence of hunting success (dens) was introduced as a factor (dens) N −1 , where N is the number of hunters at a given location. In the main simulations, density dependence was estimated as (0.9) N −1 . This produces values of daily probability of hunting success very close to what is observed in hunter-gatherers ( Table 1 ). Exploration of the parameter dens is shown in Supplementary Methods and Supplementary Fig. 7 . To simulate the age-related increase in mortality observed in humans, we used a two-parameter background daily mortality probability given by 1−exp(−( a / b ) × (exp( b × (age+1))−exp( b × (age−1)))), where age is in days, a =2.7 × 10 −7 and b =2.4 × 10 −4 . Parameters a and b were chosen so as to maximize match to published mortality curves for hunter-gatherers [45] . The chosen parameter values produce, for example, a yearly mortality rate close to 0 from age 15 to 16 years, and around 0.37 from age 70 to 71 years, independently of any energy-based considerations. Total mortality rate is background mortality multiplied by energy-dependent mortality (which can be considerably higher). Our simulations assume a number of 20 locations (location number). Each location may or may not be occupied at any given time. One of us (A.B.M.) has studied a population of 800 Agta hunter-gatherers spread around 20 camps, or an average of 40 individuals per camp. Based on Marlowe [22] , this corresponds to about seven family units per camp. Explorations of the parameter dens are shown in Supplementary Methods and Supplementary Fig. 8 . Demand sharing is mostly commonly observed in the case of large game. We therefore modelled big game hunting and the energy value of a kill k on the size of large deer, which are frequently hunted by all hunter-gatherers in Africa, Southeast Asia and America. However, k may also be seen as the value of all kills (large or small game) resulting from a hunting trip. Based on data on caloric consumption by family units, and on deer size and caloric value, we derived a value of k =4, or eight times daily caloric needs of a family unit. Hawkes et al . [46] report that Hadza hunters brought to camp a total live weight of 10,115 kg from 71 large animals, or an average of ~140 kg per carcass. About 40 kg of consumable meat can be extracted from a carcass of that size and 1 kg of meat has a caloric value of ~1,500 kcal [16] , or a total of ~60,000 kcal per deer or total acquired prey. On the other hand, the total consumption per agent or family is about 7,500 kcal (0.5 energy unit). This implies that one large deer could provide energy for approximately eight family units. For this reason, we had k =4 units from a single carcass and DCs=0.5 unit in the model. However, we also varied the parameter (see Supplementary Methods and Supplementary Fig. 9 for parameter exploration). Each agent has a level of energy, which is increased by feeding and reduced by DCs, HCs and MCs. Our agents represent family units and hence maintenance costs should reflect two adults and dependent offspring of all ages. We adopted a simplifying assumption of a fixed DC of 0.5 units (roughly 7,500 kcal per day) to reflect a lifetime average and a constant turnover of offspring growing up to independence while others are born. The daily value of 7,500 kcal per family units is not far off real estimates [16] . Explorations of the parameter DCs are shown in Supplementary Methods and Supplementary Fig. 10 . HCs include costs of hunting, transporting and processing the kill. We chose a flat value of 0.4 units (or ~6,000 kcal). Explorations of the parameter HC are shown in Supplementary Methods and Supplementary Fig. 11 . In a real setting, MCs of the agent (that is, the whole family unit) vary depending on distance between old and new location. In our model, we assume a constant cost of 0.3 units, corresponding to ~4,500 kcal. However, we have tested a range of parameter values ( Supplementary Methods and Supplementary Fig. 12 ). Agents can store up to a maximum of energy storage ( f) =15 units of energy in the form of body fat reserves in the whole family unit. This cumulative energy balance is continuously updated as a function of daily net energy income. The value of f =15 corresponds to 30 days of survival without eating, roughly corresponding to reports based on hunger strikers [47] . Beyond 30 days, survival should therefore depend on forms of storage other than body fat (such as food storage, which is not observed in simple hunter-gatherers [1] ). Explorations of the parameter f are shown in Supplementary Methods and Supplementary Fig. 13 . Agents move to another random location whenever the amount of food they obtain in a given location is not sufficient. This is achieved by equipping agents with a 3-day memory of their net energy income (a balance of energy income from hunting and sharing on the one hand and costs of hunting and maintenance on the other) at the current location, which triggers movement from a location if its mean value drops below a threshold. It should be emphasised that although movement is triggered by this 3-day net income balance (and the thresh value, death of an agent is determined by its overall (cumulative) energy balance. Measures of 3-day energy income are not limited by storage upper limits (that is, an agent with energy level near f can count all energy income regardless of whether it would take its stored energy above f ) to better reflect the quality of the environment. Agents must have been in their location for at least 2 days before they are allowed to move again to experience the new environment. Explorations of the parameter thresh are shown in Fig. 4 , Supplementary Methods and Supplementary Fig. 14 . In Supplementary Fig. 15 , we show the results for varying age at independence (age), or the age at which offspring become independent agents (that is, when they establish new family units). In our main simulations, age at independence was set at 15 years. It should be noticed that age 15 in our simulations is a minimum age for start of reproduction and not average age of first reproduction (average age of reproduction would be later, as it depends on having a high-enough energy balance, and on average our agents at age 15 years are still highly reliant on food transfer, consuming more energy than they are able to produce), see Fig. 5 . Reproduction can begin when agents become independent (at age 15 years). To reflect the costs of bringing up offspring over their dependent period, we established the conditions that reproduction is only possible if an agent has sufficient energy in the present (13.5 units, or 90% of the maximum storage level given by f =15 units), had sufficient energy over the last 15 years (also an average of 13.5 units) and has not reproduced within the last 365 days (to define an inter-birth interval reflecting human pregnancy length). There is also a random factor associated with reproduction to reduce the probability that two agents will reproduce on the same day. In our main simulations we used a RepT value set at RepT=13.5 energy units. The value represents 90% of the total storage capacity of the agent ( f =15). This indicates that the amount of body fat necessary for reproduction would have to be kept high, reflecting the expensive offspring produced by our species. Explorations of the parameter RepT are shown in Supplementary Methods and Supplementary Fig. 16 . Comparisons between simulations and real hunter-gatherers data We recorded data in our main simulations to compare with published data from hunter-gatherers. Several measures were taken on death for each individual in the model and a mean value calculated across all individuals within a replicate population. These are number of offspring, mean group size experienced, number of moves (used to calculate mean number of days between moves) and age at death (used to calculate age-specific life expectancy). Results on frequency of mobility, camp size and rates of hunting success for the simulation are reported in Table 1 , in comparison with real hunter-gatherers. Daily probability of hunting success is a product of three factors: the probability of finding food in a locality (quality of environment, p ), age-specific hunting ability and the presence of other hunters. If we assume peak hunting ability (in our model, a probability of 90% of making a kill if game is present in the locality at age 35 years) and no competition from other hunters, predicted hunting success of a peak producer is 0.9 times 0.65 (the average environmental quality in the variable environment, where p varies between 0.3 and 1), or ~58%. This value matches real data ( Table 1 ). To calculate energy income and production, data were taken from a population census on 1 day every year for the duration of the simulation ( Fig. 5 ). The age and hunting success and whether an individual hunted on that day were recorded, pooled and averaged across age categories (age<20 years, and then in decades up to the oldest living individual). Net income was plotted, having subtracted any HCs. Consumption data are measures of how much energy is available to the individuals each day, regardless of whether it is used or stored. Simulated data from five replicate populations are combined. Parameters used were as given above and an environment with a fixed probability of finding game to hunt (environmental quality) of p= 0.75. Age-specific life expectancy for simulated populations of (i) demand sharers with free riders and (ii) loners were calculated from one representative replicate for each ( Supplementary Table 1 ). Agents were censused on death, with each dead agent’s age recorded, and data were then grouped by age into decades. In simulated populations, life expectancy is calculated only for agents that survive to age at independence. Environmental quality was fixed at p= 0.75. To calculate age-specific life expectancy, the number of individuals dying within an age decade was divided by the number living to be that age and older to give mortality q x . Age-specific survival ( l x ) was calculated as the product of (1− q x ) for each x up to that age. Finally, the age specific life-expectancy ( e x ) was calculated as , where the infinite sum was taken over all remaining ages recorded (that is, to the oldest individual). Real data are from Blurton-Jones [48] for the Hadza and calculated data are from from Headland et al . [49] for the Agta. Male and female data and combined data were calculated from Hill and Hurtado [50] for the Ache and synthetic male and female data and combined data were calculated from Hill et al . [51] For the Agta, female and male life-tables contain only individuals of those sexes, whereas the combined life-tables include all individuals, irrespective of whether gender was specified. The results show that demand sharing increases life expectancy in comparison with loners, and that loners and chimpanzees show relatively similar life expectancies. How to cite this article: Lewis, H. M. et al . High mobility explains demand sharing and enforced cooperation in egalitarian hunter-gatherers. Nat. Commun. 5:5789 doi: 10.1038/ncomms6789 (2014).